Non-volatile organic memory with sub-millimetre bending radius High-performance non-volatile memory that can operate under various mechanical deformations such as bending and folding is in great demand for the future smart wearable and foldable electronics. Here we demonstrate non-volatile solution-processed ferroelectric organic field-effect transistor memories operating in p- and n-type dual mode, with excellent mechanical flexibility. Our devices contain a ferroelectric poly(vinylidene fluoride-co-trifluoroethylene) thin insulator layer and use a quinoidal oligothiophene derivative (QQT(CN)4) as organic semiconductor. Our dual-mode field-effect devices are highly reliable with data retention and endurance of >6,000 s and 100 cycles, respectively, even after 1,000 bending cycles at both extreme bending radii as low as 500 μm and with sharp folding involving inelastic deformation of the device. Nano-indentation and nano scratch studies are performed to characterize the mechanical properties of organic layers and understand the crucial role played by QQT(CN)4 on the mechanical flexibility of our devices. The realization of electronic devices that operate at extreme mechanical deformation is essential for the next generation of smart wearable and foldable electronic applications [1] , [2] , [3] , [4] . In particular, high-performance flexible non-volatile memories based on various data storage principles such as resistive type [5] , [6] , [7] , [8] , [9] , [10] , [11] , [12] , [13] , [14] , [15] , [16] , [17] , [18] , [19] , [20] , [21] , [22] , [23] , [24] , flash [4] , [25] , [26] , [27] , [28] , [29] and ferroelectric [30] , [31] , [32] , [33] , [34] , [35] , [36] , [37] , [38] , [39] , [40] hold great promise in a variety of emerging applications ranging from mobile computing to information management and communication. While the recent advances in this area are impressive, novel organic materials and electronic device structures that can be tightly rolled, crumpled, stretched, sharply folded and unfolded repeatedly without any performance degradation still need to be developed. Ferroelectric-gate field effect transistors (Fe-FETs) with ferroelectric polymer layers as gate insulators have received specific attention due to their nondestructive readout capabilities, the scalable feature size of 4F [2] and their low operating voltages [31] , [32] . In a Fe-FET, the polarity of the programme/erase gate voltage determines the polarization state of the ferroelectric layer, which in turn controls the accumulation or depletion of carriers in the semiconducting channel between the source and drain electrode, giving rise to characteristic current hysteresis [32] , [33] . To realize extremely flexible Fe-FET devices, great care should be taken in the design/selection of organic semiconductors so as to prevent the formation of cracks during and after the application of a repetitive large mechanical stress and ensure excellent adhesion properties with the ferroelectric polymer layer to avoid delamination at interfaces. Although significant progress has been made in improving certain characteristics of ferroelectric polymer memories [30] , [31] , [32] , [33] , [34] , [35] , only a few works have addressed mechanically flexible Fe-FETs in which characteristic ferroelectric switching has been examined under a relatively mild bending radius on the order of a few millimetres [36] , [37] , [38] . 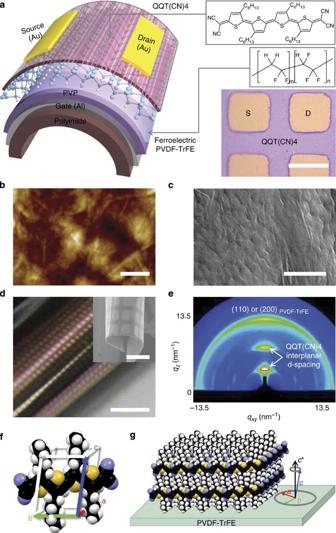Figure 1: Ultraflexible and foldable organic Fe-FET memory devices. (a) Schematic representation of the devices and molecular structure of the organic semiconductor QQT(CN)4 and the ferroelectric PVDF-TrFE. A photograph of arrays of Fe-FET devices is also displayed. Scale bar, 200 μm. (b) Height contrast TM-AFM image of a QQT(CN)4 film spin-coated onto a PVDF-TrFE layer. Scale bar, 1 μm. (c) SEM image of the surface of a QQT(CN)4 film under extreme bending. The characteristic polycrystalline texture of QQT(CN)4 was also well developed on multilayers of PVDF-TrFE/PVP/Al formed on the PI surface. Scale bar, 3 μm. (d) Photograph of arrays of flexible Fe-FET devices prepared on a PI substrate. Scale bar, 2 mm. An SEM image of extremely flexible arrays fabricated onto a paper substrate is shown in the inset. Scale bar in the inset, 500 μm. (e) 2D grazing incidence X-ray diffraction image of a PVDF-TrFE/QQT(CN)4 bilayer. (f) Illustration of QQT(CN)4 crystallographic unit cell in as-prepared film. Thick white lines indicate the triclinic 3D unit cell and the coloured arrows represent the unit cell axes. (g) Schematic representation of QQT(CN)4 molecular packing in as-prepared film on PVDF-TrFE surface and orientation of domains in the film (the black arrow points the direction of thec* axis; the coloured arrows distributing in a disc or in a cone represent the distribution of direct lattice vectors). Besides ferroelectric memories, most of the previous non-volatile memories are categorized as bendable devices when their bending radii are much greater than 1 mm ( Supplementary Table 1 ). Memories with further severe bending have rarely been demonstrated and bending radii lower than 1 mm remain exceptional, preventing rational and low-cost strategies from developing. Furthermore, no memory device has been properly operated with extreme mechanical deformation, that is, folding that resulted in permanent, plastic deformation of a device with an infinite radius of curvature at the folded line. More importantly, systematic analysis of mechanical properties of thin constituent organic and polymeric layers of a flexible device has rarely been performed. Motivated by the recent progress in the synthesis of high performance ambipolar and n-type quinoidal oligothiophene derivatives [41] , [42] , we are interested not only in employing these materials in air-stable solution-processed non-volatile memory devices applicable under such a severe mechanical deformation but also in understanding the stress relaxation mechanism of the flexible device through a new methodology used to quantify the mechanical properties of thin organic films. Herein, we report on the realization of high-performance non-volatile organic memory with excellent mechanical flexibility. The solution-processed Fe-FETs with ferroelectric poly(vinylidene fluoride-trifluoroethylene) (PVDF-TrFE) and semiconducting dicyanomethylene-substituted quinoidal quaterthiophene derivative (QQT(CN)4) exhibited p-type and n-type current hysteresis, which arises from majority carrier type conversion induced in QQT(CN)4 by a simple thermal annealing treatment [43] , [44] , [45] . In both switching modes, the memory device shows outstanding mechanical flexibility. Our Fe-FETs required no additional mechanical stress-release layers to protect the devices [3] , [46] . They are highly reliable with excellent data retention and endurance of >6,000 s and 100 cycles, respectively even after both multiple bending cycles at extreme bending radii as low as 500 μm and sharp folding involving inelastic deformation of the device. In addition to nano-indentation studies, which demonstrated that QQT(CN)4 is stiffer and more plastic than PVDF-TrFE, nano scratch experiments revealed extremely strong bonding interface between QQT(CN)4 and PVDF-TrFE. Through the stress analysis of composite films during bending, we then suggest that both the plasticity of QQT(CN)4 and its firm interface with PVDF-TrFE are responsible for resisting inelastic mechanical deformation such as folding. This work represents a major step in the development of ultraflexible organic memories and also demonstrates that solution-processed polycrystalline thin films and their interfaces can be suitably designed for extremely bendable organic electronic devices that can withstand repeatedly sharp folding and crease without suffering any degradation. Organic Fe-FET memory devices operating in dual mode Fe-FET memory devices with a bottom-gate top-contact structure consisting of an Au source–drain (S/D) electrode/solution-processed organic semiconductor/PVDF-TrFE/poly(vinyl phenol) (PVP)/Al gate electrode were constructed on either Si wafer or flexible polymer substrates, as illustrated in Fig. 1a . We employed a bilayered gate insulator composed of a ~500-nm-thick PVP dielectric layer and a 300-nm-thick PVDF-TrFE ferroelectric layer to minimize gate leakage through the ferroelectric film [47] . A solution-processable low-bandgap QQT(CN)4 with a chemical structure shown in Fig. 1a was spin-coated on the bilayer. As-prepared p-type and annealed n-type organic QQT(CN)4 FETs were previously found to exhibit hole and electron mobilities as high as 0.1 and 0.015 cm 2 V −1 s −1 , respectively ( Supplementary Fig. 1 ) [43] , [44] , [45] . These mobility values are high enough to realize ferroelectric polymer memory devices in both p- and n-type modes. Arrays of Fe-FETs were developed by thermal evaporation of Au gate electrodes, as shown in the optical microscopy (OM) image of Fig. 1a . A smooth and uniform as-prepared QQT(CN)4 layer on a PVDF-TrFE film exhibits characteristic thread-like crystals as shown in Fig. 1b . The surface morphology of this sample is similar to that previously observed in QQT(CN)4 films spin-coated onto SiO 2 (ref. 43 ). The devices fabricated on polyimide (PI) substrates are indeed extremely flexible and rollable without delamination of the components or mechanical crack formation as shown in Fig. 1c,d . Figure 1: Ultraflexible and foldable organic Fe-FET memory devices. ( a ) Schematic representation of the devices and molecular structure of the organic semiconductor QQT(CN)4 and the ferroelectric PVDF-TrFE. A photograph of arrays of Fe-FET devices is also displayed. Scale bar, 200 μm. ( b ) Height contrast TM-AFM image of a QQT(CN)4 film spin-coated onto a PVDF-TrFE layer. Scale bar, 1 μm. ( c ) SEM image of the surface of a QQT(CN)4 film under extreme bending. The characteristic polycrystalline texture of QQT(CN)4 was also well developed on multilayers of PVDF-TrFE/PVP/Al formed on the PI surface. Scale bar, 3 μm. ( d ) Photograph of arrays of flexible Fe-FET devices prepared on a PI substrate. Scale bar, 2 mm. An SEM image of extremely flexible arrays fabricated onto a paper substrate is shown in the inset. Scale bar in the inset, 500 μm. ( e ) 2D grazing incidence X-ray diffraction image of a PVDF-TrFE/QQT(CN)4 bilayer. ( f ) Illustration of QQT(CN)4 crystallographic unit cell in as-prepared film. Thick white lines indicate the triclinic 3D unit cell and the coloured arrows represent the unit cell axes. ( g ) Schematic representation of QQT(CN)4 molecular packing in as-prepared film on PVDF-TrFE surface and orientation of domains in the film (the black arrow points the direction of the c * axis; the coloured arrows distributing in a disc or in a cone represent the distribution of direct lattice vectors). Full size image The two-dimensional (2D) grazing incident X-ray diffraction (GIXD) results in Fig. 1e show the presence of both PVDF-TrFE and QQT(CN)4 crystals. In addition, no particular epitaxial crystallization could be seen on the PVDF-TrFE, meaning that the crystalline structure of the QQT(CN)4 thin films prepared on either PVDF-TrFE or SiO 2 (ref. 43 ) is similar. Crystal structure of powdered QQT(CN)4 in a triclinic system was revealed by powder X-ray experiment with help of simulated X-ray pattern analysis ( Supplementary Fig. 2 ). The detailed orientation of QQT(CN)4 crystals on PVDF-TrFE surface was obtained by extensive GIXD measurements and the results clearly show that c * axis of QQT(CN)4 crystals was preferentially aligned parallel to the surface normal as schematically illustrated in Fig. 1f . In this orientation of the crystals, flexible alkyl chains of QQT(CN)4 molecules are dominantly aligned perpendicular to the surface of PVDF-TrFE, rendering the molecules well adapted on the corrugated semi-crystalline nanostructure as schematically illustrated in Fig. 1g . The flexible alkyl chains self-assembled in between each molecular packing layer of QQT(CN)4 can be beneficial for effective release of mechanical stress upon large deformation, which is confirmed with both nano-indentation and nano scratch experiments shown later in details ( Supplementary Fig. 2 ). Before application of various mechanical stresses, we first examined memory performance of a Fe-FET with newly employed semiconductor, QQT(CN)4. As illustrated in Fig. 2a , the transfer curves (at a V DS of −5 V) of a Fe-FET with an as-prepared p-type QQT(CN)4 film present hysteresis loops arising from the ferroelectric polarization switching of the PVDF-TrFE. The sharp increase by approximately three orders of magnitude of the drain/source current ( I DS ) at negative V G originates from hole accumulation at the interface between the PVDF-TrFE and QQT(CN)4 layers. This abrupt transition corresponds to switching from the OFF state to the ON state of the memory devices and occurs when the gate field exceeds the coercive field of the ferroelectric polymer [30] . Because of the nonvolatile remnant polarization of the PVDF-TrFE layer, the I DS values remain large when V G returns to zero. 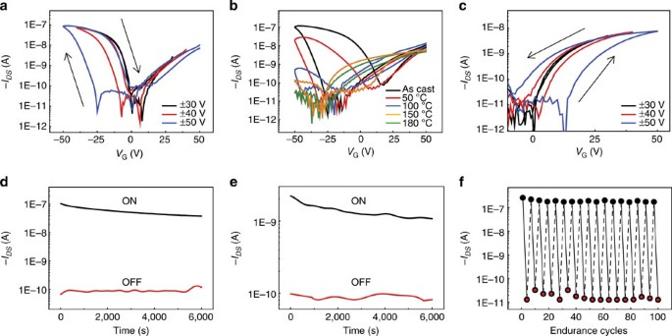Figure 2: Performance of QQT(CN)4 Fe-FET memories in p- and n-type dual mode. (a) Transfer characteristics of an as-prepared p-type QQT(CN)4 Fe-FET measured atVDS=−5 V. (b) Transfer characteristics of the QQT(CN)4 devices after annealing at different temperatures for 10 s each. (c) Transfer characteristics of an n-type QQT(CN)4 Fe-FET that was annealed at 180 °C for 10 s. The arrows show the current switching directions of the p- and n-type hysteresis curves. (d,e) Data retention characteristics measured for p-type and n-type devices, respectively, withVDS=−5 V andVDS=+5 V after programming the device with single voltage pulses for the ON and OFF current. (f) Write/erase endurance cycle test as a function of the number of programming cycles for the p-type QQT(CN)4 Fe-FETs. For clarity, one cycle out of every four is represented. The programming voltage pulses for switching ON and OFF states of a p-type Fe-FET were −50 and +50 V, respectively. The read voltages of the p-type Fe-FET for both ON and OFF states wereVG=−10 V andVDS=−5 V. The programming voltage pulses for switching ON and OFF states of an n-type Fe-FET were +50 and −50 V, respectively. The read voltages of the n-type Fe-FET for both ON and OFF states wereVG=10 V andVDS=5 V. Apparently, the memory window depends on the V G sweep range, and the best memory performance in our devices is achieved with a V G sweep of ±50 V. Figure 2: Performance of QQT(CN)4 Fe-FET memories in p- and n-type dual mode. ( a ) Transfer characteristics of an as-prepared p-type QQT(CN)4 Fe-FET measured at V DS =−5 V. ( b ) Transfer characteristics of the QQT(CN)4 devices after annealing at different temperatures for 10 s each. ( c ) Transfer characteristics of an n-type QQT(CN)4 Fe-FET that was annealed at 180 °C for 10 s. The arrows show the current switching directions of the p- and n-type hysteresis curves. ( d , e ) Data retention characteristics measured for p-type and n-type devices, respectively, with V DS =−5 V and V DS =+5 V after programming the device with single voltage pulses for the ON and OFF current. ( f ) Write/erase endurance cycle test as a function of the number of programming cycles for the p-type QQT(CN)4 Fe-FETs. For clarity, one cycle out of every four is represented. The programming voltage pulses for switching ON and OFF states of a p-type Fe-FET were −50 and +50 V, respectively. The read voltages of the p-type Fe-FET for both ON and OFF states were V G =−10 V and V DS =−5 V. The programming voltage pulses for switching ON and OFF states of an n-type Fe-FET were +50 and −50 V, respectively. The read voltages of the n-type Fe-FET for both ON and OFF states were V G =10 V and V DS =5 V. Full size image In order to transform the p-type Fe-FET into one with n-type transfer characteristics, the devices were successively annealed at increasing temperatures ranging from 50–180 °C for 10 s each. As shown in the transfer hysteresis curves of the device during successive thermal treatments in Fig. 2b , electron conduction was not strongly affected by the thermal treatment. In parallel, the hole current gradually decreased when increasing annealing temperature and time. The results obtained when switching from the OFF state to the ON state at positive V G in the devices annealed at 150 and 180 °C demonstrate that a simple thermal treatment can give rise to both p- and n-type dual-mode non-volatile Fe-FETs. In fact, fully saturated n-type current hysteresis with a gate voltage sweep of ±50 V was obtained in a Fe-FET device thermally annealed at 180 °C for 10 s, as shown in Fig. 2c . The memory device reliability of our dual mode Fe-FET was examined by both time-dependent data retention and multiple data write/erase endurance tests. The data retention properties of a Fe-FET with p-type and n-type current modulation were characterized independently by programming either an ON or OFF state once with appropriate single gate voltage pulses of ±50 V and by subsequently measuring I DS as a function of time at V DS =−5 V and V DS =+5 V, respectively. The data obtained with the p-type and n-type memories are shown in Fig. 2d,e , respectively. In both devices, the ON and OFF currents did not significantly vary even after a time period longer than 6,000 s in spite of the different ON/OFF ratios of the two devices, as dictated by the saturated curves shown in Fig. 2a,c . For multiple data write/erase endurance measurements, we consecutively read ON and OFF non-volatile I DS values with the programmed endurance cycle. In the case of the Fe-FET with p-type current modulation, very consistent and reliable rewritable endurance was observed over 100 cycles, as shown in Fig. 2f . Similar results were obtained for the device with n-type characteristics. In addition, the reversible mode switching of our Fe-FET from n-type to p- and back to n-type device was conveniently obtained by simple solvent vapour exposure. ( Supplementary Fig. 3 and Supplementary Note 1 ). It should also be noted that a very small threshold voltage shift of our Fe-FET was observed during the endurance tests. The statistical analysis of the threshold voltage shift of both turn-on and turn-off events upon repetitive write and erase endurance cycles showed the very narrow variations, within a few percentage of the total programme voltage, of both turn-on and off threshold voltages ( Supplementary Fig. 4 ). Ultraflexible organic Fe-FET memory devices Our Fe-FETs are suitable for operation under extreme mechanical stresses. We investigated the mechanical bending stability of a Fe-FET with a p-type mode on a flexible PI substrate while ON/OFF ratios were monitored as a function of the bending radius; the results are displayed in Fig. 3a . The ON/OFF ratios of the device were measured in situ at various bending states with the apparatus shown in the inset of Fig. 3a ; no significant variation in the ratios was observed. In particular, in situ current measurements were carefully performed with our super-flexible memory arrays rolled on a commercially available coffee stirrer, as illustrated in Fig. 3b . A reasonably high ON/OFF ratio of ~5 × 10 3 was obtained even at an extreme bending radius of ~500 μm. We further examined the memory stability of our Fe-FET as a function of the number of bending cycles. Both outward and inward bending were examined to evaluate the memory reliability under elongation and compression fields at the interface of the QQT(CN)4 and PVDF-TrFE layer, respectively. The device exhibited very stable ON/OFF characteristics after >1,000 bending cycles using a radius of 4 mm in both bending directions, as shown in Fig. 3c,d (also see Supplementary Figs 5 and 6 ). It should be mentioned that the minimum bending radius our automated bending cycle tester reached is 4 mm and no significant alteration in performance was observed after tens of multiple bending cycles with bending radius of ~500 μm by hand. Our p-type Fe-FET on a flexible substrate also demonstrated reliable long term data retention and multiple write/erase endurance under severe bending cycles at a radius of 4 mm, as shown in Fig. 3e,f , respectively. It is also important to emphasize that the results obtained for the n-type memories ( Supplementary Fig. 7 ) show similar outstanding mechanical stability under extreme bending conditions. 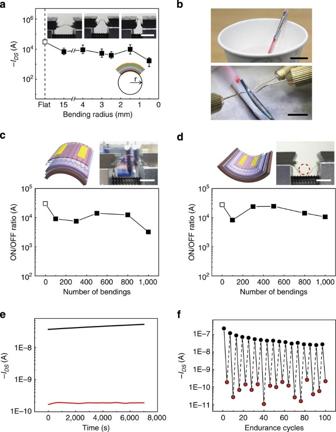Figure 3: Bending tests on ultraflexible organic Fe-FET memories. (a) ON/OFF current ratio measured atVDS=−5 V as a function of the bending radius in a p-type QQT(CN)4 Fe-FET device. The data were averaged with 10 devices examined for each bending radius. Photographs of a flexible QQT(CN)4 device at various bending states during these measurements are shown in the inset. Scale bar in the inset, 5 mm. (b) Photographs of super-flexible devices rolled on a commercially available coffee stirrer with a bending radius of ~500 μm (top image), andin situmeasurements of the rolled devices (bottom image). The scale bars of the top and bottom images are 1 cm and 5 mm, respectively. (c,d) ON/OFF current ratio measured in a p-type QQT(CN)4 Fe-FET as a function of the number of bending cycles in outward and inward directions, respectively. These measurements were performed atVDS=−5 V with a bending radius of 4 mm. The scale bars are all 1 cm. (e) Data retention characteristics measured after programming the device with single voltage pulses for the ON and OFF current in a p-type QQT(CN)4 Fe-FET after 1,000 inward bending cycles at a bending radius of 4 mm. (f) Write/erase endurance cycle test as a function of the number of programming cycles in a p-type QQT(CN)4 Fe-FET after 1,000 outward bending cycles at a bending radius of 4 mm. For clarity, one cycle out of every four is represented. The programming voltage pulses for switching ON and OFF states were −50 and +50 V, respectively. The read voltages for both ON and OFF states wereVG=−10 V andVDS=−5 V. Figure 3: Bending tests on ultraflexible organic Fe-FET memories. ( a ) ON/OFF current ratio measured at V DS =−5 V as a function of the bending radius in a p-type QQT(CN)4 Fe-FET device. The data were averaged with 10 devices examined for each bending radius. Photographs of a flexible QQT(CN)4 device at various bending states during these measurements are shown in the inset. Scale bar in the inset, 5 mm. ( b ) Photographs of super-flexible devices rolled on a commercially available coffee stirrer with a bending radius of ~500 μm (top image), and in situ measurements of the rolled devices (bottom image). The scale bars of the top and bottom images are 1 cm and 5 mm, respectively. ( c , d ) ON/OFF current ratio measured in a p-type QQT(CN)4 Fe-FET as a function of the number of bending cycles in outward and inward directions, respectively. These measurements were performed at V DS =−5 V with a bending radius of 4 mm. The scale bars are all 1 cm. ( e ) Data retention characteristics measured after programming the device with single voltage pulses for the ON and OFF current in a p-type QQT(CN)4 Fe-FET after 1,000 inward bending cycles at a bending radius of 4 mm. ( f ) Write/erase endurance cycle test as a function of the number of programming cycles in a p-type QQT(CN)4 Fe-FET after 1,000 outward bending cycles at a bending radius of 4 mm. For clarity, one cycle out of every four is represented. The programming voltage pulses for switching ON and OFF states were −50 and +50 V, respectively. The read voltages for both ON and OFF states were V G =−10 V and V DS =−5 V. Full size image Sharply foldable organic Fe-FET memory devices To further demonstrate that our Fe-FET with QQT(CN)4 can still operate properly after repetitive sharp folding actions with permanent plastic deformation of a device, arrays of devices were carefully folded so as to establish a folding line precisely located in between the source and drain electrode of a device, as shown in both OM image and schematic of Fig. 4a,b . 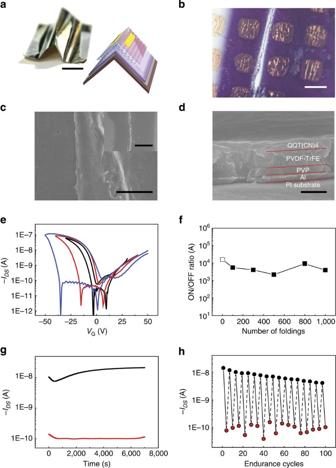Figure 4: Performance of QQT(CN)4 Fe-FET memories after sharp folding. (a) A photograph of arrays of QQT(CN)4 Fe-FET devices prepared on an Al-coated PI substrate while being sharply folded. Scale bar, 1 cm. A schematic is also shown of a device after folding in a direction of the folding-induced strain perpendicular to the source drain channel. (b) An OM image showing a deformed line arising from the folding event between source and drain electrode. Scale bar, 200 μm. (c) A SEM image of the folded line with inelastic deformation of the substrate. Scale bar, 3 μm. An inset shows a zoomed out folding line. Scale bar, 50 μm. (d) A SEM image of a cross-sectional view of a folded Fe-FET device. Scale bar, 500 nm. (e) Transfer characteristics of a p-type QQT(CN)4 Fe-FET after sharp folding. The drain voltageVDSis −5 V. (f) ON/OFF current ratio of hysteresis curve measured in a p-type QQT(CN)4 Fe-FET as a function of the number of folding cycles. (g) Data retention characteristics measured in a device after 1,000 folding cycles. The ON and OFF current were measured after programming the device with −60 and +60 V single pulses, respectively. (h) Write/erase endurance cycle test as a function of the number of programming cycles forQQT(CN)4 Fe-FET after 1,000 folding cycles. For clarity, one cycle out of every four is represented. The programming voltage pulses for switching ON and OFF states were −50 and +50 V, respectively. The read voltages for both ON and OFF states wereVG=−10 V andVDS=−5 V. Figure 4c indeed shows a sharp folding line of ~10 μm in width associated with the imposed inelastic deformation of the substrate. Interestingly, a cross-sectional image of a folded device of Fig. 4d clearly shows that all the layers that consist of the device are apparent from Al gate electrode, PVP insulator, PVDF-TrFE and QQT(CN)4 without any visible voids arising from layer delamination as further discussed later. Figure 4: Performance of QQT(CN)4 Fe-FET memories after sharp folding. ( a ) A photograph of arrays of QQT(CN)4 Fe-FET devices prepared on an Al-coated PI substrate while being sharply folded. Scale bar, 1 cm. A schematic is also shown of a device after folding in a direction of the folding-induced strain perpendicular to the source drain channel. ( b ) An OM image showing a deformed line arising from the folding event between source and drain electrode. Scale bar, 200 μm. ( c ) A SEM image of the folded line with inelastic deformation of the substrate. Scale bar, 3 μm. An inset shows a zoomed out folding line. Scale bar, 50 μm. ( d ) A SEM image of a cross-sectional view of a folded Fe-FET device. Scale bar, 500 nm. ( e ) Transfer characteristics of a p-type QQT(CN)4 Fe-FET after sharp folding. The drain voltage V DS is −5 V. ( f ) ON/OFF current ratio of hysteresis curve measured in a p-type QQT(CN)4 Fe-FET as a function of the number of folding cycles. ( g ) Data retention characteristics measured in a device after 1,000 folding cycles. The ON and OFF current were measured after programming the device with −60 and +60 V single pulses, respectively. ( h ) Write/erase endurance cycle test as a function of the number of programming cycles forQQT(CN)4 Fe-FET after 1,000 folding cycles. For clarity, one cycle out of every four is represented. The programming voltage pulses for switching ON and OFF states were −50 and +50 V, respectively. The read voltages for both ON and OFF states were V G =−10 V and V DS =−5 V. Full size image The deformed device still displayed characteristic ferroelectric hysteresis fully saturated with a V G of approximately ± 60 V with ON/OFF current ratio similar to that obtained before folding test ( Supplementary Fig. 8a ), as shown in Fig. 4e . In addition, reliable ON and OFF current retention and rewritable endurance were observed with respect to time over 7,000 s. and over 100 cycles, respectively ( Supplementary Fig. 9 ). The device also exhibited very stable ON/OFF characteristics after >1,000 folding cycles, as shown in Fig. 4f (see also Supplementary Fig. 8 ). The highly reliable retention and rewritable endurance of our device were well preserved even after 1,000 folding cycles as shown in Fig. 4g,h , respectively. Field effect mobility of the folded device was ~0.08 cm 2 V −1 s −1 , very similar to the one obtained before folding. Our results clearly indicate that the electrical properties of both the QQT(CN)4 and ferroelectric PVDF-TrFE layers have not been altered with permanent plastic deformation. Our foldable memory was also prepared on commercially available chewing gum aluminium paper ( Supplementary Fig. 10 ). Again, the Al paper with arrays of Fe-FETs was carefully folded to make a folded line developed in between the source and drain electrode of a device. Similar to the results of a memory on PI substrate, the deformed device exhibited characteristic ferroelectric hysteresis with reliable ON and OFF current retention ( Supplementary Fig. 10 ). Although intrinsic switching of a PVDF-TrFE involving the rotation of H-F dipole around C–C backbone occurred in approximately a few nano-second levels, its switching speed can vary, depending on the types of devices [48] . For instance, field effect transistor type devices exhibited switching time of 10 −3 to 10 −4 s, irrespective of organic semiconductors with their field effect mobilities ranging from 0.05 to ~1 cm 2 V −1 s −1 (refs 49 , 50 , 51 ). Our Fe-FET with p-type QQT(CN)4 having the field effect mobility of ~0.1 cm 2 V −1 s −1 would certainly show the switching behaviour similar to those from previous works. The literature suggests that our FET device can be useful for an application requiring kHz-level frequency operation. This range of switching speed is highly relevant to applications of growing interest such as flexible electronic papers and books. High ON/OFF ratio is also one of the important factors that should be considered. In most of OFETs with relatively low-mobility organic semiconductors, the ON/OFF ratio can significantly be enhanced by the reducing OFF current level, which is sensitive to gate leakage current. It is also true in principle for non-volatile memory applications that higher the ON/OFF ratio, better is the device performance. The accepted minimum ON/OFF margin for proper memory operation is, however, set ~100 and sometimes the margin of 10-fold difference can be allowed. While the strategy herein presented should be applicable to other materials and guide the design of novel materials, lowering the voltage operation of our device remains challenging mainly due to the many structural defects and large surface roughness of the PVDF-TrFE insulator layer. A thick ferroelectric gate insulator is indeed often required to minimize the electric leakage as we have shown in our device, resulting in high operating gate voltage greater than 50 V. However, to successfully demonstrate a low-voltage operation of our Fe-FET, instead of using a PVP layer to reduce gate leakage, we newly employed a novel nanocomposite interlayer consisting of chemically reduced graphene oxides homogeneously embedded in an insulating polymer. Ultra-thin dielectric polymer interlayer with conductive 2D materials was expected to effectively reduce the operation voltage. The preliminary results indeed show a Fe-FET with the interlayer operated at 25 V ( Supplementary Fig. 11 and Supplementary Note 2 ) with reliable memory retention and write/erase endurance cycles. More systematic studies are under way. Since ferroelectric PVDF-TrFE is very tolerant to mechanical stimuli such as extension and compression ( Supplementary Fig. 12 ), the excellent memory performance of our Fe-FETs after severe bending and folding deformation apparently strongly relies on the mechanical properties of QQT(CN)4 thin films, as well as the interfacial properties between PVDF-TrFE and QQT(CN)4. Considering further the molecular packing of QQT(CN)4 ( Fig. 1e ), we associate the flexible alkyl chains grafted to the quinoidal oligothiophene backbone with the film’s ability to compensate for the strain [52] , [53] . The outstanding mechanical stability of the crystalline QQT(CN)4 thin films arises from conformal deposition of oligomeric QQT(CN)4 molecules on the PVDF-TrFE layer. The latter consists of surface-corrugated, needle-like crystalline domains with dimensions of ~200 nm × 40 nm, which leads to excellent adhesion of the QQT(CN)4 film, then, sustaining extreme mechanical stresses. Furthermore, these flexible alkyl chains grafted to the quinoidal oligothiophene backbone preferentially align normal to the interface ( Fig. 1g and Supplementary Fig. 2c ), allowing the easy sliding of packed molecular sheets of QQT(CN)4 with each other, and compensating the strain built up in the film. The surface morphology of the flexible Fe-FET device after severe bending cycles was not different from that before mechanical stress was applied, and no cracks or degradation of the thin QQT(CN)4 film were observed. In addition, no delamination of the composed layers occurred. Fine mechanical cracks aligned parallel to the bending plane were observed only on the surface of the Au source and drain electrodes ( Supplementary Fig. 13 ). Even after folding deformation, there was no fracture on QQT(CN)4 except numerous wrinkled lines arising from the plastic deformation as also evidenced by the cross-sectional view of a folded device in Fig. 4d ( Supplementary Fig. 14 ). The two effects of (1) the easy molecular adaptation of QQT(CN)4 layer to the corrugated PVDF-TrFE crystalline surface and (2) the bi-layered structure with the characteristic mechanical properties of PVDF-TrFE and QQT(CN)4 were combined with each other and gave rise to a novel non-volatile polymer memory device even with permanent deformation of the channel after folding. To fully apprehend the importance of the role of QQT(CN)4 and its interplay with the PVDF-TrFE layer, it is important to note that devices based on 6,13-Bis (triisopropylsilylethynyl) pentacene (TIPS-PEN), poly (3 hexyl thiophene) (P3HT) and 5,11-Bis (triethylsilylethynyl) anthradithiophene (TES-ADT) did not work after both bending and sharp folding ( Supplementary Fig. 15 ). These results do emphasize how the mechanical properties of QQT(CN)4 are truly remarkable. The detailed mechanical properties of the thin layers are examined next. Mechanical properties of a PVDF-TrFE/QQT(CN)4 bilayer In order to understand the mechanical behaviours of our devices, we characterized the mechanical properties of PVDF-TrFE and QQT(CN)4 on PVDF-TrFE by nano-indentation. We also used this technique to measure the mechanical properties of commercially available semiconductor films including P3HT, TIPS-Pentacene and TES-ADT for comparison purposes. Samples with ~300-nm-thick PVDF-TrFE, ~100-nm-thick QQT(CN)4 film on ~300-nm-thick PVDF-TrFE, and ~100-nm thick other organic semiconductor films on ~300-nm-thick PVDF-TrFE were prepared on Si substrates. We tried to have films with the same thickness. However, it was difficult to fabricate a QQT(CN)4 film thicker than 100 nm due to the limited solubility of this compound and the low viscosity of the QQT(CN)4 solution arising from its low molecular weight. Representative indentation curves for PVDF-TrFE, QQT(CN)4/PVDF-TrFE and P3HT/PVDF-TrFE are presented in Fig. 5a . Instrumented tests were completed and, using both the maximum applied load and the given penetration depth in the indentation curves, the hardness, H IT , was calculated. We found that H IT for PVDF-TrFE, QQT(CN)4/PVDF-TrFE and P3HT/PVDF-TrFE are very similar, yielding values of 126.6±6.4 MPa, 144.2±13.9 MPa and 140.8±6.2 MPa, respectively ( Fig. 5b ). The elastic modulus, noted E IT , was obtained from the slope of unloading curve in the indentation experiment. The E IT values for PVDF-TrFE, QQT(CN)4/PVDF-TrFE and P3HT/PVDF-TrFE were estimated to be 7.8±0.2 GPa, 12.8±1.0 GPa and 11.5±0.6 GPa, respectively ( Fig. 5b ). 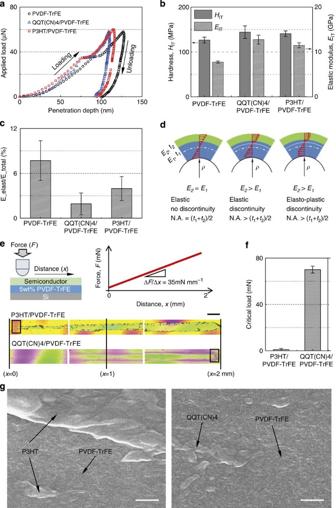Figure 5: Characterization of the mechanical properties by nano-indentation and nano scratch test. (a) Representative loading and unloading curves in nano-indentation tests. (b) An instrumented testing hardness,HIT, and an instrumented testing elastic modulus,EITfor PVDF-TrFE, QQT(CN)4 coating on PVDF-TrFE and P3HT coating on PVDF-TrFE. Each bar is an average value with s.d. for five indentation tests. (c) The ratio of elastic energy (Eelast) to the total energy (Etotal) for PVDF-TrFE, QQT(CN)4 coating on PVDF-TrFE and P3HT coating on PVDF-TrFE. Each bar is an average value with s.d. for five indentation tests. (d) Schematic of bending stress distribution of a two-layered film under the condition of elastic deformation withE2=E1, elastic deformation withE2>E1, and elasto-plastic deformation withE2>E1at the same radius of curvatureρ(centroid of geometry (dot-dashed line), neutral axis, N.A. (dotted line), Young’s modulus (E1) and thickness (t1) of substrate, and Young’s modulus (E2) and thickness (t2) of top layer). (e) Schematic of nano scratch test with a ramp loading and representative optical images along the scratches after tests for P3HT coating on PVDF-TrFE and QQT(CN)4 coating on PVDF-TrFE. A rectangular box in the image indicates a region where a critical load is defined. Scale bar, 50 μm. (f) Critical loads for P3HT/PVDF-TrFE and QQT(CN)4/PVDF-TrFE bilayers. Each bar is an average value with s.d. for five nano scratch tests. (g) The magnified SEM images taken at the region of the rectangular box in (e). As denoted by arrows, semiconductor coatings (P3HT and QQT(CN)4) and the underlying layer of PVDF-TrFE can be readily identified in the images. Scale bar, 300 nm. Figure 5: Characterization of the mechanical properties by nano-indentation and nano scratch test. ( a ) Representative loading and unloading curves in nano-indentation tests. ( b ) An instrumented testing hardness, H IT , and an instrumented testing elastic modulus, E IT for PVDF-TrFE, QQT(CN)4 coating on PVDF-TrFE and P3HT coating on PVDF-TrFE. Each bar is an average value with s.d. for five indentation tests. ( c ) The ratio of elastic energy ( E elast ) to the total energy ( E total ) for PVDF-TrFE, QQT(CN)4 coating on PVDF-TrFE and P3HT coating on PVDF-TrFE. Each bar is an average value with s.d. for five indentation tests. ( d ) Schematic of bending stress distribution of a two-layered film under the condition of elastic deformation with E 2 = E 1 , elastic deformation with E 2 > E 1 , and elasto-plastic deformation with E 2 > E 1 at the same radius of curvature ρ (centroid of geometry (dot-dashed line), neutral axis, N.A. (dotted line), Young’s modulus ( E 1 ) and thickness ( t 1 ) of substrate, and Young’s modulus ( E 2 ) and thickness ( t 2 ) of top layer). ( e ) Schematic of nano scratch test with a ramp loading and representative optical images along the scratches after tests for P3HT coating on PVDF-TrFE and QQT(CN)4 coating on PVDF-TrFE. A rectangular box in the image indicates a region where a critical load is defined. Scale bar, 50 μm. ( f ) Critical loads for P3HT/PVDF-TrFE and QQT(CN)4/PVDF-TrFE bilayers. Each bar is an average value with s.d. for five nano scratch tests. ( g ) The magnified SEM images taken at the region of the rectangular box in ( e ). As denoted by arrows, semiconductor coatings (P3HT and QQT(CN)4) and the underlying layer of PVDF-TrFE can be readily identified in the images. Scale bar, 300 nm. Full size image To investigate the effect of underlying substrate Si on measurements, indentation tests were performed at various loads. We have found that the estimated values of H IT and E IT for PVDF-TrFE barely change when the penetration depth is <150 nm, corresponding to 50% of the film thickness ( Supplementary Fig. 16 and Supplementary Note 3 ). We note that the value of E IT estimated at the minimum penetration depth by our indentation method is quite similar to the one obtained from the buckling experiments [54] . E IT for QQT(CN)4 is ~64% higher than that for PVDF-TrFE, although their H IT values are similar. As E IT is estimated from the slope of elastic recovery during unloading, the difference in E IT might be attributed to a degree of elastic deformation. In this regard, we calculated the ratio of elastic energy to the total energy by dividing the area under the unloading curve by the area under the loading curve ( Fig. 5c ). Compared with PVDF-TrFE and P3HT, the ratio for QQT(CN)4 is significantly low, which indicates that the material behaviour of QQT(CN)4 is more plastic than elastic. This result accounts for the morphology of QQT(CN)4 layer after folding, containing many wrinkled lines ( Supplementary Fig. 14 ). To understand how mechanical bending of a composite film depends on material properties and to clarify the role played by the mechanical behaviour of QQT(CN)4, we developed a model based on a bi-layer film as shown in Fig. 5d . We analysed the normal stress distribution inside the film with parameters obtained from experiments such as film thickness and Young’s modulus of PVDF-TrFE and QQT(CN)4, assuming that it undergoes a pure bending. The difference of material properties between QQT(CN)4 and PVDF-TrFE causes the neutral axis to move away from the centroid of geometry and the normal stress to become discontinuous at the interface between the two layers. If QQT(CN)4 is nine times stiffer than PVDF-TrFE, the neutral axis is located at the interface and therefore the stress at the interface becomes zero ( Supplementary Fig. 17 and Supplementary Note 4 ). According to our experimental results, the ratio of Young’s modulus for QQT(CN)4 to PVDF-TrFE is 1.6. This suggests that the neutral axis is located at 221 nm from the bottom of the PVDF-TrFE layer. The average stress at the interface is then similar to the case when the stiffness of QQT(CN)4 and PDVF-TrFE is identical ( Supplementary Fig. 17 and Note 4 ). In addition, plastic characteristic of QQT(CN)4 can form a more complex stress distribution. When the applied moment produces a stress that exceeds a yield stress, stress will remain constant or barely change in the region of plastic deformation in contrary to the linearly varying stress observed in purely elastic materials. The stress analysis implies that the QQT(CN)4 layer helps to reduce the stress and strain at the interface by putting the neutral axis close to it, and to keep the maximum stress relatively low with plastic deformation. The interfacial properties of semiconductor/PVDF-TrFE bilayers were also important for maintaining memory performance under bending and folding. Therefore, adhesion between layers were extensively examined by nano scratch experiments as well as layer delamination tests with commercially available Scotch tapes. The delamination experiments clearly showed that the interface of QQT(CN)4 and PVDF-TrFE was very firm while interfaces of other semi-conductors examined with PVDF-TrFE were not robust as shown in Supplementary Fig. 18 and Supplementary Note 5 . However, such a crude delamination test was not sufficiently accurate to quantify the interfacial strength of the bilayers. For a more quantitative analysis of the interfacial properties of the films, we developed a modified nano scratch technique. In these experiments, the adhesion strength of organic semi-conductor/PVDF-TrFE bilayers was successfully estimated using a stainless steel ball in contact with a bilayer. With an increasing mechanical force, a line was drawn at constant speed ( Fig. 5e ). Critical load values were identified at failure of the semiconductor layers ( Fig. 5f ). It should be noted that unlike common nano scratch tests where few micrometre-sized tips were used for the measurements, a stainless steel ball with 1.6-mm diameter was used to produce the contact pressure suitable for observing failure at the interface between the semiconductor coatings and PVDF-TrFE films. The ramp loading, from 1 mN to 70 mN, was applied on the ball while tangentially moving of 2 mm at a speed of 2 mm min −1 to determine the critical load when the organic semiconductor coatings are mostly delaminated and PVDF-TrFE film started to appear due to the large contact stress. Tearing of the film at failure was confirmed by visualizing the scratched surface using scanning electron microscopy ( Fig. 5g , Supplementary Fig. 19c and Supplementary Note 6 ). The results of critical load demonstrate the extremely firm interface between QQT(CN)4 and PVDF-TrFE, compared with those of other bilayers ( Supplementary Fig. 19a and Supplementary Note 6 ). This convincingly explains the effective mechanical stress release upon severe deformation observed with QQT(CN)4. To further confirm the crucial role of QQT(CN)4 with fluorinated polymer having semi-crystalline nanostructure, we employed another fluorinated polymer, poly(vinylidenefluoride- co -trifluoroethylene- co -chlorotrifluoroethylene) (PVDF-TrFE-CTFE), which has the similar crystalline surface structure to PVDF-TrFE ( Supplementary Fig. 20a ). Owing to its relaxer characteristics with nearly zero remnant polarization as well as with its large electrostrictive strain of a few percents, a device fabricated with the terpolymer exhibited excellent p-type switching behaviour instead of non-volatile memory performance. ( Supplementary Fig. 20b ) The switching properties of the device were well maintained under repetitive folding deformation. ( Supplementary Fig. 20c and d ) No significant delamination was observed in the nano scratch test, suggesting that QQT(CN)4 and PVDF-TrFE-CTFE form a stable interface. ( Supplementary Fig. 20e ) The results imply again that strong adhesive properties of QQT(CN)4 with PVDF-TrFE were responsible for maintaining the high performance under the deformation in our device. Previous studies have demonstrated polymeric solar cells and light-emitting diodes with an unprecedented mechanical flexibility and an ability to be stretched [55] , [56] . These devices could still operate properly for radii of curvatures as low as 10 μm and was found to be stretch-compatible to 100% tensile strain. In case of small molecule-based organic electronic devices, bending radii of 100 μm or less and stretchability have been also achieved but an encapsulation layer was needed to place the active organic films near the neutral plane position [3] , [46] . With no additional mechanical stress-release layers, the most flexible organic field-effect transistors based on a polycrystalline organic semiconducting layer could be bent without any degradation of their electrical performance to a radius as low as 260 μm (ref. 57 ). Although degradation of these devices based on bis-(triisopropylsilylethynyl) pentacene or bis-triethylsilylethynyl anthradithiophene thin films was observed below a critical bending radius of ~200 μm, these results provided evidence that crystalline solution-processed organic semiconducting materials could be intrinsically more flexible than initially thought. In that context, our study demonstrates p- and n-type dual-mode organic Fe-FET memories with highly reliable data retention and endurance and, more importantly, with outstanding mechanical flexibility. It should be emphasized that our devices can be sharply folded and creased repeatedly without the need of using an encapsulation layer to protect them against mechanical damage. The evidence that polycrystalline organic electronic layers and their interfaces can withstand such extreme mechanical strains without suffering any degradation represents an important milestone in the field of organic electronics. The outstanding mechanical flexibility of our devices are essentially due to the remarkable mechanical properties of QQT(CN)4 as demonstrated by our nano-indentation and nano scratch study. This work should represent an important step towards the design and the development of novel solution-processable organic-conjugated materials combining enhanced mechanical flexibility with excellent semiconducting properties. We have herein identified essential features associated with the molecular structures of both the quinoidal QQT(CN)4 and fluorinated polymers. The results suggest that for extreme mechanical stresses to be sustained a corrugated polymer surface with nanometre-scale crystalline domains is important as it can lead to an excellent adhesion of the semiconductor layer. Flexible alkyl chains should preferentially align normal to the interface with the base polymer. This crystalline organisation allows for easy sliding of packed molecular sheets with one another, which then compensate the strain built up in the film. The presence of side chains is certainly not sufficient, as demonstrated when comparing results obtained with QQT(CN)4 and P3HT. Then, small molecules appear to bear a strong advantage as demonstrated by the critical load results, which explains the effective mechanical stress release upon severe deformation. In conclusion, we develop a high-performance air-stable non-volatile Fe-FET memory operating in p- and n-type dual modes with excellent mechanical flexibility. In both non-destructive carrier-type modes, the device with solution-processed polycrystalline multiple layers exhibits excellent data retention and endurance of >6,000 s and 100 cycles, respectively. Furthermore, our Fe-FETs are found to be highly robust towards severe mechanical stimuli such as bending and sharp folding, even without the use of an additional device protection treatment. No significant performance degradation is observed at repetitive extreme bending events with the bending radii as low as 500 μm or even after 1,000 folding cycles involving inelastic deformation of the device. Mechanical tests using nano-indentation and nano scratch techniques reveal that the stable performance at large strains is due to the plastic characteristics of QQT(CN)4 and firm interface between the polycrystalline PVDF-TrFE and QQT(CN)4 layers. Our p- and n-type dual-mode foldable Fe-FETs significantly outrun other memory devices previously reported in terms of mechanical flexibility. These results could offer a new strategy for low-power consumption organic CMOS circuits combining outstanding mechanical flexibility with logic and memory functionalities. In addition, our study shows that not only polymers but also polycrystalline solution-processed organic thin films and their interfaces, if carefully designed, can withstand extreme mechanical deformation without any degradation, which is essential for the future development of foldable and stretchable organic electronic applications. Materials and device fabrication PVDF-TrFE with 25 wt% TrFE was purchased from MSI Sensors. QQT(CN)4 was synthesized following an improved method adapted from the literature [44] . P3HT ( M W =180,000 g mol −1 with 98.5% head-to-tail regio-regularity), TIPS-PEN (99.9% purity) and TES-ADT (99% purity) were purchased from Sigma-Aldrich, Korea. All organic solvents, including methyl ethyl ketone (MEK), were purchased from Sigma Aldrich. Si substrates were cleaned in successive ultrasonic baths of acetone and ethanol for 1 h each, while the PI and Al paper substrates with the thickness of ~0.1 mm and 0.02 mm, respectively used for the flexible devices were sonicated only in ethanol for 2 h. For the devices prepared on PI sheets, bottom aluminium gate electrodes of ~100 nm in thickness were thermally evaporated through a shadow mask onto the substrate under a vacuum of 10 −6 Torr (SNTEK MEP5000). Poly(4-vinyl phenol) (PVP), PVDF-TrFE and QQT(CN)4 layers were then prepared sequentially from solution by spin-coating. The PVP films were prepared from a solution in propylene glycol monomethyl ether acetate (PGMEA) and then baked at 200 °C for 30 min. The ferroelectric copolymer PVDF-TrFE films were deposited from a MEK solution and dried in vacuum at 135 °C for 2 h. PVDF-TrFE-CTFE films were deposited from a 5 wt% solution in MEK and dried in vacuum at 135 °C for 2 h. As-prepared p-type QQT(CN)4 thin films were spin-coated from chloroform. To achieve a majority carrier type conversion from p-type to n-type, the films were annealed on a hot plate at 180 °C for 10 s. 1 wt% P3HT solutions in DCB were spin-coated at a spin rate of 2,000 r.p.m. for 1 min. 1 wt% TIPS-PEN solutions in toluene were spin-coated at a spin rate of 2,000 r.p.m. for 1 min. 4 wt% TES-ADT solutions in toluene were spin-coated at a spin rate of 1,500 r.p.m. for 1 min. All solutions were used after filtration with 1 μm PTFE membrane. As-prepared p-type QQT(CN)4 thin films were spin-coated from chloroform. To achieve a majority carrier-type conversion from p-type to n-type, the films were annealed on a hot plate at 180 °C for 10 s. To complete the device fabrication procedure, arrays of top-contact 30 nm-thick Au source/drain electrodes were thermally evaporated through a shadow mask under a vacuum of 10 −6 Torr. The channel width and length of our devices were ~200 and 100 μm, respectively. Note that the fabrication of our devices was carried out in ambient atmosphere. Device characterization The electrical characteristics of our devices were measured using a probe station and a semiconductor analyser system (E5270B, Agilent Technologies) under ambient conditions. Field emission scanning electron microscopy (FESEM) images were acquired using a LEO 1550 VP with an acceleration voltage of 15 kV and no metal deposition. Atomic force microscopy (AFM) measurements were carried out using a Digital Instruments NanoScope 3100 microscope. An optical microscope (Olympus BX 51 M) was also employed to visualize the Fe-FET devices. 2D grazing incidence X-ray diffraction experiments were performed at the Pohang Accelerator Laboratory in Korea. The films were placed on an x - and y -axis goniometer and irradiated with monochromatized X-rays ( λ =0.10608, nm) having grazing incidence angles ranging from 0.09° to 0.15°. The scattered beam intensity was measured with an SCX:4300-165/2 CCD detector (Princeton Instruments). A powder X-ray diffraction pattern of QQT(CN)4 was recorded at 300 K in transmission mode (0.3 mm dia. capillary; synchrotron radiation, λ =0.099939, nm; 2 θ range: 3.0–70.0; step width: 0.01° on a diffractometer equipped with an imaging plate detector at the RIKEN Materials Science Beamline (BL44B2) at SPring-8 (ref. 58 ) Structure was solved by a simulated annealing method with the programme DASH [59] . The obtained structure was refined with Rietveld method with the programme RIETAN-FP [60] . Restraints but no constraints for all bond lengths were employed to maintain the molecular geometry. Thermal temperature factors were refined isotropically, and uniform values were applied. Final Rietveld refinement: a =8.0471(3), b =9.8417(5), c =14.7557(5) Å, α =102.056(5), β =98.903(4), γ =98.754(3)°, V =1108(2) Å 3 (ref. 60 ), R wp =3.09% ( R e =1.92%), R p =2.29%, R B =4.40% and R F =3.94%. We characterized the material properties of PVDF-TrFE, QQT(CN)4, and other semiconductor films on Si substrates by using nano-indentation technique (CSM Instrument, Switzerland). It should be noted that the maximum penetration depth should be as shallow as possible in order to avoid the substrate effect. To this end, the penetration depths were measured with the minimum applied force of ~60 μN on the Berkovich tip with loading and unloading speed of 60 μN min −1 . Mechanical properties were obtained from simple interpretation of the indentation curves by using Oliver–Pharr method [61] , [62] , [63] . The modified nano scratch test (CSM Instrument, Switzerland) was conducted on various bilayers by displacing a 1.6 mm dia. stainless steel ball at a speed of 2 mm min −1 with an increasing load from 1 mN to 70 mN. From the images with optical microscope and SEM, critical loads when the semiconductor coatings are mostly delaminated and a PVDF-TrFE film starts to appear were determined. How to cite this article: Kim, R. H. et al. Non-volatile organic memory with sub-millimetre bending radius. Nat. Commun. 5:3583 doi: 10.1038/ncomms4583 (2014).